Single-male paternity in coelacanths Latimeria chalumnae , a ‘living fossil,’ is of great scientific interest, as it is closely related to the aquatic ancestors of land-living tetrapods. Latimeria show internal fertilization and bear live young, but their reproductive behaviour is poorly known. Here we present for the first time a paternity analysis of the only available material from gravid females and their offspring. We genotype two L. chalumnae females and their unborn brood for 14 microsatellite loci. We find that the embryos are closely related to each other and never show more than three different alleles per locus, providing evidence for a single father siring all of the offspring. We reconstruct the father’s genotype but cannot identify it in the population. These data suggest that coelacanths have a monogamous mating system and that individual relatedness is not important for mate choice. Coelacanths, an ancient lineage of fish, were thought to be extinct for more than 60 mya until Marjorie Courtenay-Latimer discovered an individual on a fishing trawler in 1938 later to be scientifically described as Latimeria chalumnae [1] . As this very first report from South Africa, more than a hundred individuals have been found off the East African Coast, most of them on the Comoros [2] , [3] . Researchers refer to coelacanths as ‘living fossils’ because of their nearly unchanged morphology since the late Devonian, approximately 400 mya ago [4] . They are of major scientific interest as they represent a very basal group of the gnathostomes. Consequently, a lot of studies investigated the phylogenetic relationship between coelacanths, lungfish and tetrapods [5] , [6] , [7] , [8] . Also, the divergence of the two coelacanth species L. chalumnae in Africa and Latimeria menadoensis in Indonesia has attracted quite a lot of scientific attention [9] , [10] , [11] , [12] . The nearly unchanged morphology of coelacanths for the last 400 mya [4] , [13] has led to the conclusion that their behaviour, ecology and genetics are very likely unchanged since the Devonian, and several molecular studies have confirmed their slow rate of evolution at the genetic level [14] , [15] , [16] , [17] . However, recent population genetic studies revealed genetic divergence between individuals among and within the field sites and thus a potential for adaptation in L. chalumnae [18] , [19] . Still they present an opportunity to get fascinating insights into the ecology and behaviour of a very old animal group. Because they have such a high scientific value, coelacanth ecology has been studied quite extensively despite their relatively secluded habitat. Several studies on coelacanth biology have revealed many details about their life histories and ecology. We know that Latimeria occurs in water depths below 100 m (refs 20 , 21 , 22 ). They prefer caves to rest during the day [23] , [24] . They are active at night and ambush predators but have a very low metabolic rate probably allowing for long periods without food [25] . Coelacanths have rather large home ranges, but low dispersal rates and population sizes seem small [20] , [23] , [26] . In fact, despite their ability to adapt to different habitats, there is no doubt that Latimeria has to be considered a rare and an endangered species [20] , [27] . As presented, L. chalumnae is quite an extensively studied species; however, a lot of questions remain, so far, unresolved. For example, free swimming juveniles are rarely seen and do not live together with the adults, leading to the assumption that they withdraw to other habitats possibly to escape cannibalistic adults [28] , [29] . Also, the reproductive behaviour of coelacanths is largely unknown. 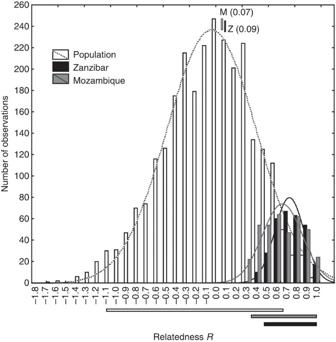Figure 1: Distribution of individual relatedness. The distribution ofRvalues and 95% confidence intervals (bars below the graph) are given for the total population (light bars;n=70) ofLatimeria chalumnaeand within the clutches (Zanzibar–black bar (n=23); Mozambique–grey bar (n=26)). The relatedness values of the parents of both clutches are given (values in brackets) and their position within the relatedness values of the total population is shown (black bar–Z=Zanzibar parents; grey bar–M=Mozambique parents). The capture of gravid females with full-term embryos ( Table 1 ) has proven that L. chalumnae are ovoviviparous and give birth to live young [30] , [31] . Embryos have large yolk sacs that are retained almost until birth. Morphological structures to directly nurture the embryo (exclusively or in addition to the maternally provisioned yolk) have so far not been discovered [28] , [31] , [32] , [33] . The period of embryogenesis is estimated to last approximately 3 years [20] meaning a very large investment for the female carrying the young. The internal fertilization, necessary for intrauterine development of the eggs, however, functions without externally visible copulatory organs. Male L. chalumnae might possess a cloaca [34] that could even be used as an eversible copulatory organ [31] ; however, matings have so far never been observed and even the existence of the cloaca has been debated [35] . Table 1 List of all documented cases of gravid Latimeria chalumnae *. Full size table The absence of external copulatory organs means that females cannot easily be forced into copulations [36] . As females invest a lot of time and energy into each clutch, it seems likely that they should optimize the offsprings’ fitness by being selective about their mating partners. Females might even choose to mate with several mates to ensure fertilization of the full clutch, to enhance the genetic variability of the offspring or to make sure that the fittest male sires her clutch. In this paper, we present the first molecular analyses of gravid females and their offspring. We use microsatellites to investigate the genetic diversity of the two only available coelacanth broods. We find a low genotypic variability and high relatedness of the offspring of each female. We show that each clutch was sired by a single male, with no evidence for multiple paternities. From reconstruction of the paternal genotypes, we show that females do not use relatedness criteria (preference or avoidance of closely related individuals for mating) for mate choice. Genetic diversity Embryos in both females were well developed and seemed close to being born soon. Both females had roughly the same number of embryos: 26 (CCC 162–Mozambique) and 23 (CCC 253– Zanzibar). In both clutches, a maximum of three alleles per locus are found. Mean homozygosity per locus (HL) is very similar in all groups: full population HL=0.47±0.20 s.d., Mozambique HL=0.46±0.15 s.d., Zanzibar HL=0.42±0.17 s.d.). Consequently, no significant difference is detected between the groups (ANOVA: SQ=0.059, FG=2, MQ=0.029, F =0.895, P =0.411). In the 26 Mozambique embryos, 22 different genotypes were identified all of which were different from the maternal genotype. Four genotypes were represented by two individuals each ( Table 2 ). This was most likely due to the very close relatedness of the siblings and relatively low marker resolution. Similarly, in the 23 Zanzibar embryos, 19 different genotypes could be identified, also all of them being different from the maternal genotype. Again, four genotypes were present, each in two different individuals ( Table 3 ). Table 2 Genotypes in family 1 (Mozambique)*. Full size table Table 3 Genotypes in family 2 (Zanzibar)*. Full size table The levels of relatedness within the clutches are very high (Mozambique R =0.60±0.23; Zanzibar R =0.68±0.15 mean±s.d.). Not surprisingly, they are significantly higher than the level of relatedness over the entire Latimeria population ( R =−0.121±0.45 mean±s.d.) (ANOVA results: SQ=310.7, FG=2, MQ=155.3, F =902.4, P <0.001; a Scheffé post hoc test reveals a significant difference between the overall population and the clutches) ( Fig. 1 ). Figure 1: Distribution of individual relatedness. The distribution of R values and 95% confidence intervals (bars below the graph) are given for the total population (light bars; n =70) of Latimeria chalumnae and within the clutches (Zanzibar–black bar ( n =23); Mozambique–grey bar ( n =26)). The relatedness values of the parents of both clutches are given (values in brackets) and their position within the relatedness values of the total population is shown (black bar–Z=Zanzibar parents; grey bar–M=Mozambique parents). Full size image Paternity analysis The low number of alleles per locus and the high level of individual relatedness within the broods indicate a single father for each clutch. This hypothesis is confirmed by the programme GERUD that calculated that a single male could have sired all offspring within each clutch. The reconstructed male genotypes were compared with all genotypes from our whole-population data set using the programme COLONY but could not be identified within the sample. For both clutches, the most closely related genotypes to the fathers’ are found to be from the Comoros. The reconstructed male from the Mozambique clutch share 11 alleles at 7 loci with an individual found at the Comoros ( R =0.211). The reconstructed male of the Zanzibar clutch is closely related ( R =0.45) to a different animal from the Comoros. Their genotypes share 14 alleles at 9 loci. The parents of both clutches are not more closely or less related to each other than the rest of the population ( Fig. 1 ). Phylogenetically, the occurrence of viviparity in coelacanths is very interesting. Although it is generally assumed that viviparity has evolved several times independently within the fishes [37] , recent findings of viviparity being widespread in placoderms [38] might suggest that internal fertilization and the bearing of live young rather was the ancestral state for all gnathostomes [39] and was lost rather than gained during evolution. At least the strategy of producing young with large yolk provisions rather than very many small eggs seems to be at least as old as 300 million years, as it has been reported also from the Carboniferous coelacanth Rhabdoderma [29] . Like every other ecological trait, the internal fertilization and development of juveniles has costs as well as benefits. The main advantage of internal development, of course, is the enhancement of offspring survival. The main disadvantage of internal embryonic development is the increased costs of reproduction per individual offspring for the female. Females suffer reduced fecundity and might even face higher predation pressure due to lower mobility during pregnancy [40] , [41] . In coelacanths, the benefits of live-bearing seem to compensate the large disadvantages to the female. Even though an estimated 3-year developmental phase [28] means a great investment into each embryo from the mother, this might be advantageous as the offspring might escape cannibalistic attacks from adults [29] . Another interesting aspect of the bearing of live young is the internal fertilization mode in coelacanths. Internal fertilization without copulatory organs is rare among the viviparous fishes but can be found, for example, in the Goodeidae [42] (even though they do have a differentiated anal fin [43] ). Coelacanths completely lack external copulatory organs or even modified structures, although they clearly have internal fertilization. For a mating to be successful even without male copulatory organs, matching body sizes of the mating partners seem to be the key factor that influences the reproductive output to a great amount [42] . All these considerations (high maternal costs per offspring, fertilization rate correlated to morphology) lead to the conclusion that females should choose their mating partners very carefully to optimize the offspring number and survival. Multiple mating seemed as a way to ensure the highest potential level of successful fertilization, the highest level of genetic variability in the offspring as well as ensuring the inheritance of the best genes in the offspring [44] . However, contrary to our expectations, both investigated clutches were clearly sired by a single male. Even though sample size is low, this finding might indicate that coelacanths have a monogamous mating system. Monogamous mating systems are most commonly found in species where the father also provides parental care or where there is no opportunity for polygamy [45] . As in coelacanths, we have no information about any parental care after birth. It seems more likely that females do not mate multiply, because they do not have the opportunity or because multiple matings do not provide enough benefits to outweigh the potential costs. Potential costs to multiple mating could be the enhanced energy expense needed to search for mates and the potentially enhanced predation and infection risks during mating and mate search. Another very interesting finding of our study was the relatedness pattern found between parents: mother and father of a clutch were not closer or had less relatedness than the majority of random pairs of the Latimeria population. This might mean that females avoid mating with close relatives; however, it could also mean that mating occurs randomly with respect to the overall genotypic relatedness. Either the probability to meet a close relative for mating is very low [46] or other male traits might be more important than relatedness, for example, morphology (see above) or parasite resistance. The absence of female choice based on relatedness could mean that in coelacanths, no mechanism for kin recognition is implemented. This in turn would facilitate the occurrence of cannibalism (see above), which seems to be a realistic threat to juvenile Latimeria and might be the reason for the evolution of viviparity as well as behavioural adaptations in the group. In conclusion, we found that L. chalumnae juveniles are very closely related to each other and their genotypes could be explained by assuming that they were sired by a single male. Coelacanths therefore appear to present a monogamous mating system. The relatedness pattern of the parents seemed random and did not convey evidence for genetically based female choice. Due to their mating system, morphological traits could be more important for the reproductive success. This study provided new insights into coelacanth reproductive behaviour and therefore proved once more how extraordinary these animals are. Samples We used material from a female L. chalumnae , which was captured in 1991 off the coast of Mozambique. This female was found to be pregnant with 26 fully developed embryos. We also secured material from a second pregnant female that was captured in 2009 in Zanzibar bearing 23 late-term embryos ( Table 1 ). Molecular analyses We extracted DNA from all embryos and both mothers using a 20% Chelex solution protocol [47] and genotyped the samples for 14 nuclear microsatellite markers [17] , [18] . We performed PCR reactions in a total volume of 10 μl, with 1 × buffer, 1.5 mM MgCl 2 , 0.2 mM of each dNTP, 0.2 μM of each primer ( Table 4 ) and 0.05 U Taq polymerase (EuroTaq – BioCat, Heidelberg, Germany). PCR conditions were set to 5 min of denaturing at 95 °C, 40 cycles of denaturing at 95 °C for 30 s, 30-s primer specific annealing temperature (50 °C–MS2; 52 °C–MS4; 54 °C–MS1, MS7, MS10; 56 °C–MS3, MS5, GTH06; 60 °C MS6, MS8, MS11, MS18; 62 °C–MS14, MS16) and 72 °C for 30-s extension, followed by a final extension of 5 min at 72 °C. For locus GTH06, we adapted a M13 protocol. We added the M13-tail (5′-CACGACGTTGTAAAACGAC-3′) to the 5′ end of the reverse primer. Primer concentrations were GTH06F – 10 pmol, M13 primer with 800 nm fluorescent label 10 pmol and GTH06_Rtailed 2.5 pmol μl −1 ). PCR products were analysed on a Licor 4300 DNA Analyser (Licor Biosciences, Lincoln, USA). Genotyping was done using the programme Saga2 (Licor Biosciences, Lincoln, USA). In addition, we visually inspected allele sizes and corrected them manually if necessary. Table 4 Primers used for microsatellite genotyping. Full size table We analysed the Mozambique clutch using the full set of 14 microsatellites ( Table 2 ). We genotyped 11 of the 14 loci for individuals from Zanzibar (no data could be obtained from MS1, MS7 and MS10) ( Table 3 ). For the comparison to our dataset of adult individuals ( N =70) representing the entire known Latimeria chalumnae population 10 MS loci could be considered. Statistical analyses We counted the number of alleles and genotypes in the clutches. We reconstructed paternal genotypes using the programme GERUD [48] and searched for the genotypes in the reference population using the programme COLONY [49] . We calculated individual relatedness and homozygosity levels per locus using the programme STORM [50] . We compared Latimeria clutches to an already available data set of adult L. chalumnae individuals from the east coast of Africa [18] . We used STATISTICA (StatSoft Inc., Tulsa, USA) to compare the groups (ANOVA) and to produce graphs (histograms). How to cite this article: Lampert, K. P. et al. Single-male paternity in coelacanths. Nat. Commun. 4:2488 doi: 10.1038/ncomms3488 (2013).